Activation of diverse signalling pathways by oncogenicPIK3CAmutations The PIK3CA gene is frequently mutated in human cancers. Here we carry out a SILAC-based quantitative phosphoproteomic analysis using isogenic knockin cell lines containing ‘driver’ oncogenic mutations of PIK3CA to dissect the signalling mechanisms responsible for oncogenic phenotypes induced by mutant PIK3CA . From 8,075 unique phosphopeptides identified, we observe that aberrant activation of PI3K pathway leads to increased phosphorylation of a surprisingly wide variety of kinases and downstream signalling networks. Here, by integrating phosphoproteomic data with human protein microarray-based AKT1 kinase assays, we discover and validate six novel AKT1 substrates, including cortactin. Through mutagenesis studies, we demonstrate that phosphorylation of cortactin by AKT1 is important for mutant PI3K-enhanced cell migration and invasion. Our study describes a quantitative and global approach for identifying mutation-specific signalling events and for discovering novel signalling molecules as readouts of pathway activation or potential therapeutic targets. The p110α catalytic subunit of phosphatidylinositol 3-kinase (PI3K) is encoded by PIK3CA , one of the most frequently mutated genes in human cancers. Recent studies have shown that three activating mutations, E542K and E545K in the helical domain and H1047R in the kinase domain, can lead to downstream activation of PDK1 and/or AKT to promote carcinogenesis and metastasis [1] , [2] , [3] . Studies have also suggested that mutations in the kinase or helical domains have distinct effects on PI3K downstream signalling events. Zhao and Vogt [4] showed that binding to p85, the regulatory subunit of PI3K, is essential for the transformation induced by the kinase domain PIK3CA mutant (H1047R) but not for the one bearing mutations in the helical domain (E542K and E545K). A more recent study further demonstrated that the helical domain mutant, but not the kinase domain mutant, could directly associate with insulin receptor substrate 1 without the mediation of p85, which is required for activation of wild-type PIK3CA or PIK3CA with kinase domain mutations [5] . Clinical studies have shown that tumours with H1047R mutation exhibit a better response to PI3K/mammalian target of rapamycin (mTOR) inhibitors in comparison with those carrying helical domain mutations [6] , [7] . To dissect the signalling mechanisms underlying the mutant PIK3CA- induced transformation, through genetic engineering, we have developed a series of human cell lines that differ only in their PIK3CA allele status, containing either the wild-type (wt) or mutant forms of PIK3CA at codon 545 or 1,047 (refs 8 , 9 ). Both of these PIK3CA mutations can activate multiple downstream pathways, which confer the ability for growth factor-independent proliferation in vitro and metastatic capability in vivo [8] , [9] . We have also previously developed J124 as a novel and specific inhibitor of PIK3CA activity [10] . Treatment with this inhibitor can dramatically reduce AKT activity and inhibit metastasis of cancer cells bearing PIK3CA mutations. In this study, we performed phosphoproteomic analysis of a spontaneously immortalized non-tumorigenic breast epithelial cell line MCF10A along with two isogenic derivatives generated by knock-in of mutant alleles—one bearing the E545K mutation located in the helical domain in exon 9 and the other bearing the H1047R mutation located in the kinase domain in exon 20 of the PIK3CA gene (hereafter referred to as Ex9-KI and Ex20-KI) [8] . Mass spectrometry-based phosphoproteomics has become a powerful tool for studying signalling networks in a global manner, especially in conjunction with stable isotope labelling by amino acids in cell culture (SILAC) for a precise quantitative readout [11] , [12] , [13] , [14] , [15] . Here we identify and quantify 8,075 phosphopeptides, of which 1,142 are more phosphorylated in PIK3CA mutant cells and undergo a decrease in their phosphorylation status when treated with J124, a specific inhibitor of PIK3CA gene product. We use protein microarrays as a complementary platform to validate direct AKT1 substrates in vitro . Integration of the data from phosphoproteomic analysis with that from protein microarrays led to identification of a number of previously uncharacterized signalling molecules that appear to be involved in oncogenic signalling mediated through mutation of PIK3CA . Most notably, our studies identify cortactin as a novel AKT1 substrate whose phosphorylation enhances migration and invasion, key downstream events of the PIK3CA and AKT1 activation. Phosphoproteomic analysis of mutant PIK3CA knockin cells Although many studies have associated PIK3CA mutations with features of transformation, a global and quantitative study of how mutant PIK3CA impacts the signalling networks and consequently transforms epithelial cells has not yet been described. The isogenic knockin system along with a novel PIK3CA-specific inhibitor and high-resolution mass spectrometry-based quantitative phosphoproteomics provide the tools to map the signal transduction pathways that are specifically modulated by PIK3CA mutations in a comprehensive manner. To validate this system, we first examined the phosphorylation levels of AKT1 and mitogen-activated protein kinase (MAPK) in the mutant cells where we found phospho-AKT and phospho-MAPK levels to be dramatically elevated in both cells and substantially suppressed by J124 treatment ( Fig. 1a ). 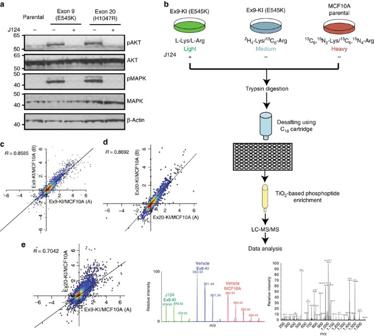Figure 1: Phosphoproteomic analysis of MCF10A cells withPIK3CAmutations. (a) Western blot analysis of phosphorylated AKT (pT308), total AKT, phosphorylated p42/44 MAPK (pThr202/Tyr204) and total p42/44 MAPK in MCF10A parental cells, Ex9-KI and Ex20-KI cells with or without J124 treatment. (b) A schematic depicting the strategy used for quantitative phosphoproteomic profiling ofPIK3CAEx9 knockin mutant cells. (c,d) Density scatter plot of log2-transformed phosphopeptide ratios (Ex9-KI or Ex20-KI versus MCF10A) from two SILAC reverse-labelled biological replicates. (e) Density scatter plot of log2-transformed phosphopeptide ratios (xaxis: Ex9-KI versus MCF10A andyaxis: Ex20-KI versus MCF10A). Pearson coefficient correlation (R) is indicated. Figure 1: Phosphoproteomic analysis of MCF10A cells with PIK3CA mutations. ( a ) Western blot analysis of phosphorylated AKT (pT308), total AKT, phosphorylated p42/44 MAPK (pThr202/Tyr204) and total p42/44 MAPK in MCF10A parental cells, Ex9-KI and Ex20-KI cells with or without J124 treatment. ( b ) A schematic depicting the strategy used for quantitative phosphoproteomic profiling of PIK3CA Ex9 knockin mutant cells. ( c , d ) Density scatter plot of log 2 -transformed phosphopeptide ratios (Ex9-KI or Ex20-KI versus MCF10A) from two SILAC reverse-labelled biological replicates. ( e ) Density scatter plot of log 2 -transformed phosphopeptide ratios ( x axis: Ex9-KI versus MCF10A and y axis: Ex20-KI versus MCF10A). Pearson coefficient correlation ( R ) is indicated. Full size image To interrogate the aberrant signalling triggered by the mutations in PIK3CA , we combined SILAC and TiO 2 -based phosphopeptide enrichment followed by liquid chromatography tandem mass spectrometry (LC-MS/MS) analysis. Lysates of MCF10A parental cells were mixed with Ex9-KI cells that were treated with vehicle or J124 in a 3-plex SILAC experiment ( Fig. 1b ). The same experimental strategy was employed for the analysis of Ex20-KI cells in a separate 3-plex SILAC experiment ( Supplementary Fig. 1b ). After enrichment of phosphopeptides with TiO 2 beads, the samples were desalted and analysed on a high-resolution Fourier transform mass spectrometer. We also carried out replicate experiments in which the SILAC labels were swapped. In all, we identified 8,075 unique phosphopeptides derived from 2,016 proteins ( Supplementary Data 1 and 2 ). Of these, 7,199 phosphopeptides harboured serine phosphorylation, 1,631 phosphopeptides contained threonine phosphorylation and 168 phosphopeptides harboured tyrosine phosphorylation, and most of the phosphopeptides were singly or doubly phosphorylated ( Supplementary Fig. 1c,d ). The SILAC ratios (KI cells versus MCF10A) of phosphopeptides obtained from the two replicate experiments of both PIK3CA knockin cells showed a strong positive correlation (the correlation coefficient R =0.86 for Ex9-KI group and R =0.87 for the Ex20-KI group) for two independent biological replicates ( Fig. 1c,d ). There were 2,469 phosphopeptides that were detected in common in the Ex9-KI and Ex20-KI experimental groups, and the SILAC ratios (Ex9-KI or Ex20-KI cells versus MCF10A) of these phosphopeptides in the two cells with PIK3CA mutations were also quite correlated ( R =0.70) ( Fig. 1e ). Of the 2,469 phosphopeptides detected in common, 826 peptides derived from 338 proteins demonstrated the same increased or decreased phosphorylation pattern (>1.5-fold change in phosphopeptide intensity for both Ex9-KI and Ex20-KI cells) when compared with MCF10A cells ( Supplementary Data 3 ). However, we also found that 417 peptides from 243 proteins were highly phosphorylated (>1.5-fold change) only in Ex9-KI ( Supplementary Data 4 ) or Ex20-KI ( Supplementary Data 5 ) cells compared with MCF10A cells, but not in both. These changes in phosphorylation patterns suggest that although downstream signalling effects are largely similar for these two particular mutant forms of PIK3CA , there are also some that are unique to the individual PIK3CA mutations. For instance, we found three kinases, PAK2, PAK4 and SLK, that were highly phosphorylated only in Ex9-KI cells and have been reported to be activated by PI3K-AKT pathway to promote cell migration/invasion [16] , [17] , [18] . It has been shown that breast cancer cells expressing PIK3CA with helical domain (Ex9) mutation are more invasive than the cells expressing PIK3CA with kinase domain (Ex20) mutations [19] , which is consistent with the data from this isogenic knockin system. The evidence of increased phosphorylation of these kinases specific to each knockin mutant cell could shed new light on some of the mechanisms underlying the phenotypic differences induced by PIK3CA Ex9 or Ex20 mutants. Global elevation of protein phosphorylation by mutant PIK3CA Overall, we observed that introduction of a single oncogenic amino acid change (E545K or H1047R) in PIK3CA can substantially elevate protein phosphorylation levels. In both Ex9-KI and Ex20-KI experimental groups, four major regulation patterns were observed. The first pattern included phosphopeptides identified in the Ex9-KI experimental group and in Ex20-KI group whose phosphorylation levels were 1.5-fold higher in mutant cells than parental cells and exhibited at least a 33% reduction in Ex9-KI/Ex20-KI cells on treatment with J124 ( Fig. 2a and Supplementary Fig. 2a ). A second pattern included peptides that were highly phosphorylated in Ex9-KI/Ex20-KI but were not substantially altered on treatment with J124 ( Fig. 2b and Supplementary Fig. 2b ). A third pattern was of peptides that were less phosphorylated in Ex9-KI/Ex20-KI but were not substantially altered on treatment with J124 ( Fig. 2c and Supplementary Fig. 2c ). The fourth pattern included a set of phosphopeptides whose phosphorylation levels were unaltered in knockin cells but underwent suppression on J124 treatment ( Fig. 2d and Supplementary Fig. 2d ). 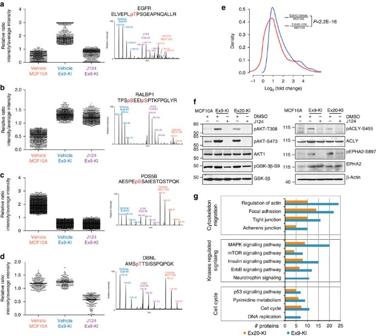Figure 2: Phosphorylation regulation patterns in MCF10A, Ex9-KI and J124-treated Ex9-KI cells. (a–d) Representative MS spectra of modulated phosphopeptides corresponding to each regulation pattern type are shown along with the phosphopeptide sequences. (e) Distribution of log2-transformed intensity ratios of phosphorylation increased peptides (Ex9-KI versus MCF10A, fold change >1.5). Thexaxis shows log2-transformed phosphopeptide intensity ratios and theyaxis shows the density. Blue represents the ratios of Ex9-KI to MCF10A cells, while red represents the ratio of J124-treated Ex9-KI to MCF10A cells. TheP-value calculated using a paired Student’st-test comparing the two distributions was 2.2E−16. (f) Western blottings to confirm the phosphorylation status of a subset of phosphoproteins using phospho-specific antibodies, along with western blottings using antibodies against total proteins. β-Actin served as loading control. (g) The number of regulated proteins found in enriched signalling pathways (Modified Fisher’s exactP-value <0.05) are shown for three biological processes—cytoskeleton and migration, kinase-regulated signalling and cell cycle. Figure 2: Phosphorylation regulation patterns in MCF10A, Ex9-KI and J124-treated Ex9-KI cells. ( a – d ) Representative MS spectra of modulated phosphopeptides corresponding to each regulation pattern type are shown along with the phosphopeptide sequences. ( e ) Distribution of log 2 -transformed intensity ratios of phosphorylation increased peptides (Ex9-KI versus MCF10A, fold change >1.5). The x axis shows log 2 -transformed phosphopeptide intensity ratios and the y axis shows the density. Blue represents the ratios of Ex9-KI to MCF10A cells, while red represents the ratio of J124-treated Ex9-KI to MCF10A cells. The P -value calculated using a paired Student’s t -test comparing the two distributions was 2.2E−16. ( f ) Western blottings to confirm the phosphorylation status of a subset of phosphoproteins using phospho-specific antibodies, along with western blottings using antibodies against total proteins. β-Actin served as loading control. ( g ) The number of regulated proteins found in enriched signalling pathways (Modified Fisher’s exact P -value <0.05) are shown for three biological processes—cytoskeleton and migration, kinase-regulated signalling and cell cycle. Full size image Overall, as compared with MCF10A cells, we observed increased phosphorylation of about 47% and 33% of peptides in Ex9-KI and Ex20-KI cells, respectively. To examine the effects of J124 on global protein phosphorylation, we generated an intensity plot depicting the distribution of log 2 -transformed intensity ratios of highly phosphorylated peptides in Ex9-KI cells versus MCF10A cells, or J124-treated Ex9-KI cells versus MCF10A cells ( Fig. 2e ). We observed that J124 treatment resulted in a significantly global shift of phosphorylation pattern in Ex9-KI cells and significantly reduced the phosphorylation levels of highly phosphorylated peptides identified in this study. A similar trend was observed in the case of Ex20-KI cells. This global trend was confirmed by western blot analysis using phospho-specific antibodies targeting some of the well-known key molecules downstream of the PI3K signalling pathway, including AKT1 and GSK3β and recently identified AKT1 substrates, ATP citrate lyase (ACLY) [20] , [21] and EPHA2 (ref. 22 ), which were elevated in knockin cells and were efficiently suppressed by J124 treatment ( Fig. 2f ). These results clearly demonstrate that activation of mutated PIK3CA leads to a global increase in protein phosphorylation and profoundly affects signalling networks. Activation of multiple signalling pathways by mutant PIK3CA To better understand the global phosphorylation alterations induced by oncogenic PIK3CA mutations, we performed a Kyoto Encyclopedia of Genes and Genomes pathway analysis using an integrated online functional annotation tool, DAVID [23] , for the proteins with increased phosphorylation in Ex9-KI and Ex20-KI cells. Representative signalling pathways that were significantly enriched ( P <0.05) in PIK3CA mutant knockin cells and involved in the biological processes, including cytoskeleton and migration, kinase-regulated signalling and cell cycle regulation are shown in Fig. 2g . In agreement with our previously reported observations [8] , our global phosphoproteomic study revealed that multiple oncogenic kinase-regulated signalling pathways such as MAPK, mTOR and ErbB were highly phosphorylated and enriched in PIK3CA mutant knockin cells. We also observed that multiple cell cycle-related pathways were enriched in mutant knockin cells, which has been previously suggested to provide a proliferative advantage in basal cell culture medium [8] . Notably, one of the pathways among the cell cycle- and cell proliferation-related pathways pertains to pyrimidine metabolism. The link between activation of PI3K-AKT pathway and regulation of pyrimidine metabolism has been described in two recent studies [24] , [25] . These studies demonstrated that mTOR signalling downstream of PI3K-AKT module could enhance the de novo pyrimidine synthesis through phosphorylation of Ser1859 on CAD (carbamoyl-phosphate synthetase 2, aspartate transcarbamylase and dihydroorotase), a site that was also detected as highly phosphorylated in our experiments. We also observed increased phosphorylation of four other key enzymes (CTPS, RRM2, TK1 and DUT), which are involved in pyrimidine metabolism ( Supplementary Fig. 4a ). Finally, pathways regulating cell migration and invasion, such as those mediating actin rearrangements, cell adhesion and tight junction networks, were also found to be enriched ( Fig. 2g and Supplementary Fig. 2e ). Widespread modulation of phosphorylation of the kinome Of the 972 proteins that were found to be highly phosphorylated by one or both PIK3CA mutants, 46 were protein kinases. Of these protein kinases, 39 and 30 kinases were highly phosphorylated at serine/threonine residues in Ex9-KI or Ex20-KI cells, respectively (22 in common), suggesting that PI3K has a broad role in regulating cellular protein kinase activity. To obtain a systematic view of these differentially phosphorylated kinases, we mapped them and the corresponding phosphorylation sites onto a phylogenetic tree of the human kinome ( Fig. 3a and Supplementary Fig. 3 ). Many of these modulated kinases have been shown to be associated with oncogenic transformation or metastasis in diverse cancers. Of the 39 highly phosphorylated kinases detected in Ex9-KI cells, elevation in the phosphorylation level of 25 kinases could be reversed by a short treatment with J124, suggesting that these kinases are likely to be directly regulated by AKT and/or PDK. Consistent with this suggestion, increased phosphorylation of S21 on GSK3A, S9 on GSK3B and S897 on EPHA2 is already known to be directly phosphorylated by AKT [22] , [26] , [27] and phosphorylation of these sites is critical in regulation of their kinase activities [19] , [22] , [23] . For instance, AKT has been recently shown to phosphorylate EPHA2 to induce ligand-independent activation of EPHA2 and to promote cell migration and invasion [22] . In addition to increased phosphorylation of receptor tyrosine kinases, such as EGFR (T693) and EPHA2 (S897), we also observed increased phosphorylation on of a non-receptor tyrosine kinase, PTK2 (S932) also known as FAK1. 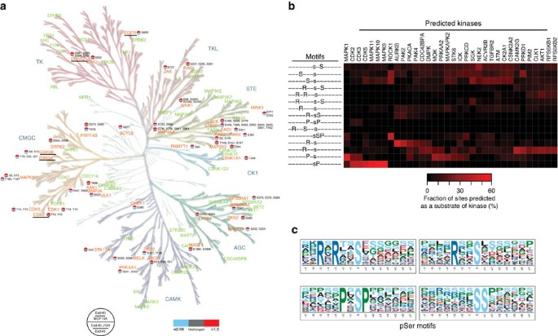Figure 3: Widespread modulation of the kinome byPIK3CAmutants. (a) A phylogenetic tree (modified from Human Kinome Tree58) of protein kinases identified in Ex9-KI cells. Phosphorylation increased kinases are in orange and kinases identified but did not change in phosphorylation levels are in light green. A colour-coded site regulation pattern is shown in the form of a circle divided into two parts. The top half represents the fold change of phosphorylation sites identified in Ex9-KI cells compared with MCF10A, whereas the bottom half represents the fold change ratio between J124-treated Ex9-KI cells compared with untreated cells. Regulated kinases that are known to be AKT substrates are underlined. (b) Significantly overrepresented linear phosphorylation motifs identified using Motif X programme were indicated on the left of the panel. Phosphopeptides matching the motifs were used for prediction of their upstream kinases by NetworKIN programme. Based on the total number of phospho-modulated peptides, percentage of the number of phosphopeptides as substrates of predicted kinases were calculated and demonstrated in the heatmap (right panel). (c) Sequence logos of overrepresented phosphoserine linear motifs enriched among the peptides whose phosphorylation levels were increased in Ex9-KI and/or Ex20-KI cells as compared with MCF10A cells. Figure 3: Widespread modulation of the kinome by PIK3CA mutants. ( a ) A phylogenetic tree (modified from Human Kinome Tree [58] ) of protein kinases identified in Ex9-KI cells. Phosphorylation increased kinases are in orange and kinases identified but did not change in phosphorylation levels are in light green. A colour-coded site regulation pattern is shown in the form of a circle divided into two parts. The top half represents the fold change of phosphorylation sites identified in Ex9-KI cells compared with MCF10A, whereas the bottom half represents the fold change ratio between J124-treated Ex9-KI cells compared with untreated cells. Regulated kinases that are known to be AKT substrates are underlined. ( b ) Significantly overrepresented linear phosphorylation motifs identified using Motif X programme were indicated on the left of the panel. Phosphopeptides matching the motifs were used for prediction of their upstream kinases by NetworKIN programme. Based on the total number of phospho-modulated peptides, percentage of the number of phosphopeptides as substrates of predicted kinases were calculated and demonstrated in the heatmap (right panel). ( c ) Sequence logos of overrepresented phosphoserine linear motifs enriched among the peptides whose phosphorylation levels were increased in Ex9-KI and/or Ex20-KI cells as compared with MCF10A cells. Full size image Phosphorylation motifs enriched in mutant PIK3CA cells The preference of amino acid motifs surrounding the phosphorylation sites is one of the major mechanisms that contribute to kinase specificity [28] . Identification of overrepresented motifs could help pinpoint upstream kinases activated by mutant PIK3CA . To determine which linear motifs were overrepresented in our data set, we used the motif-X algorithm ( Fig. 3b,c ). The peptides whose phosphorylation was increased in Ex9-KI and Ex20-KI cells and reduced on treatment with J124 were selected for this analysis. We identified 15 significantly enriched pS motifs ( Fig. 3b ) and the sequence logos of top four enriched motifs are depicted in Fig. 3c . Among these enriched motifs, eight were basic-rich motifs while three resembled the minimal AKT substrate motifs (RxRxxpS or RxxpS), which were ranked as the top two enriched phosphorylation motifs by motif-X analysis and Fig. 3c . Prediction of the kinases upstream of these regulated phosphopeptides using the NetworKIN algorithm led to identification of 34 kinases. The fraction of phosphopeptides corresponding to substrate motifs of each kinase was calculated and plotted in a heat map ( Fig. 3b ). In agreement with the results of analysis with motif-X, the AKT kinase family was predicted to target the basic-rich motifs that were enriched in our data set ( Fig. 3b ). In the integrated heat map combining motif-X and NetworKIN analysis, we observed that a large number of phosphopeptides contained sequence motifs that could be phosphorylated by RPS6K, a kinase downstream of mTOR, indicating activation of the canonical pathway from PI3K to AKT-mTOR-RPS6K. The activation of RPS6K is also supported by the fact that several phosphorylation-regulated sites known to be specifically phosphorylated by RPS6K were identified to be highly phosphorylated in PIK3CA mutant knockin cells. They are RPS6 S235/S240, EIF4B S442, HSPB1 S78/S82 and NCBP1 S22/T21. We also observed that CDK and MAPK kinases were predicted as the activated upstream kinases phosphorylating the peptides with the PxpSP substrate motif, ( Fig. 3b,c ), consistent with our previous report [8] that MAPK1 and MAPK3 were highly phosphorylated and activated in mutant PIK3CA knockin cells ( Fig. 1a ). More importantly, of these upstream kinases, 11 (MAP4K4, MAPK1, PAK2, PAK4, PRKAA1, PRKCD, RPS6KA1, CDK2, CDK3, CSNK1A1 and AKT1) were indeed found to be more phosphorylated in PIK3CA mutant cells and were downregulated upon J124 treatment ( Supplementary Data 1 ). In addition to the activation of canonical kinases (such as AKT1, RPS6K1 and MAPK1) by oncogenic PIK3CA mutations, identification of a broader spectrum of PI3K-modulated kinases, including PAK2/4, CASNK1A1, MAP4K4 and PRKCD, could bring new insights into the understanding of the mechanisms of oncogenic transformation induced by mutant PIK3CA . Interactome analysis to identify activated kinase pathways Our motif analysis indicated that kinases, including AKT, MAPKs and CDKs, were activated in PIK3CA mutant knockin cells. To understand the signalling networks more fully, we decided to study the kinase–substrate relationships and protein–protein interactions among the identified phosphoproteins. To do so, we first generated a database by integrating three kinase–substrate databases, HPRD [29] , PhosphoSitePlus [30] and Phospho.ELM [31] , with a protein–protein interaction database [32] , which merges protein–protein interaction information obtained from well-known interaction databases, including HPRD [29] , BIND [33] and IntAct [34] . After removing redundant entries, the final integrated database had 7,047 kinase–substrate pairs with 77,176 protein–protein interaction pairs. Next, we mapped 474 proteins whose phosphorylations were increased in PIK3CA mutant knockin cells and decreased on the treatment of J124, to our integrated protein–protein interaction networks. We identified 108 kinase–substrate and 310 protein–protein interaction pairs composed of 208 differentially phosphorylated proteins. There were 11 kinases that were regulated by PI3K but not mapped in the network ( Supplementary Data 6 ). The main interaction networks were visualized using Cytoscape ( Supplementary Fig. 4b ). We then used a graph theoretic algorithm, molecular complex detection, to discover highly connected interaction clusters [35] . In Fig. 4 , four of the top ranked interaction clusters are shown. Of note, in agreement with our phosphomotif enrichment analysis, phosphorylated MAPK1 and AKT1 ( Fig. 4a,b ) form the central hubs of the two top-ranked networks. This suggests not only that AKT1 and MAPK1 kinases were activated by oncogenic PIK3CA mutations, but also that their downstream proteins/targets were consequently modulated by increased phosphorylation. 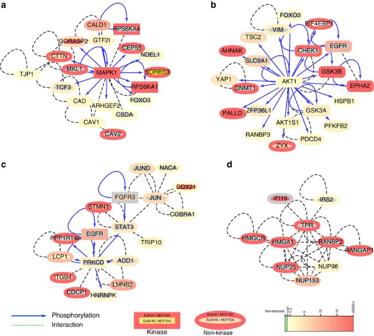Figure 4: Kinase–substrate and protein–protein interaction networks. The top four highly connected clusters that are highlighted on the main network map (Supplementary Fig. 4b) with dark green circles: (a) MAPK, (b) AKT and (c) PRKCD centred kinase–substrate and protein–protein interaction clusters. (d) The cluster enriched with NPC proteins. The network of kinase–substrate and protein–protein interaction within stringently regulated phosphoproteins was generated using Cytoscape. Proteins are colour-coded based on their ratios (Ex9-KI versus MCF10A cells outer circle and Ex20-KI versus MCF10A inner circle) of phosphosites. Figure 4: Kinase–substrate and protein–protein interaction networks. The top four highly connected clusters that are highlighted on the main network map ( Supplementary Fig. 4b ) with dark green circles: ( a ) MAPK, ( b ) AKT and ( c ) PRKCD centred kinase–substrate and protein–protein interaction clusters. ( d ) The cluster enriched with NPC proteins. The network of kinase–substrate and protein–protein interaction within stringently regulated phosphoproteins was generated using Cytoscape. Proteins are colour-coded based on their ratios (Ex9-KI versus MCF10A cells outer circle and Ex20-KI versus MCF10A inner circle) of phosphosites. Full size image In addition to these canonical pathways, there were two other clusters in the regulated phosphoprotein network. One of them is centred around PRKCD, also known as protein kinase C-δ a ubiquitously expressed isoform of the novel protein kinase Cfamily ( Fig. 4c ). This kinase can regulate apoptosis in a cell type and stimulus-dependent manner [36] . The stability and activity of PRKCD has been shown to be increased by PDK1, a key kinase in the PI3K pathway [37] . The activity of PRKCD is regulated by phosphorylation on several sites—in this study, we identified two PRKCD phosphorylation sites, S202 and S204, which were tightly correlated with PI3K activity but not well characterized previously. Of note, the amino acid sequence adjacent to Ser204 phosphorylation site matches the minimal AKT substrate motif (RxxpS), suggesting that AKT1 could potentially directly regulate PRKCD through phosphorylation. The other cluster comprises ten nuclear proteins, of which six are either known components of the nuclear pore complex (NPC) or proteins associated with the complex ( Fig. 4d ). In addition, we also detected ten other NPC or NPC-associated proteins, eight of which were highly phosphorylated in Ex9-KI and/or Ex20-KI cells ( Supplementary Fig. 4c ). Of these PI3K-regulated phosphoproteins, multiple phosphosites identified in this study have also been identified in other contexts. For instance, phosphorylation of NUP98 S591, S595 and S606 by CDK1 or NEK6 is crucial for disassembly of the NPC during mitosis [38] . Although its phosphorylation is not directly involved in NPC disassembly, RanGAP1 S428/442 is also a substrate for CDK1 (ref. 39 ). Nup153 S516, which we identified to be regulated by PI3K, was one of multiple ERK1 phosphorylation sites identified in this protein [40] . ERK1 phosphorylation of Nup153 decreased recognition of a nuclear transport receptor. We also identified phosphorylation of RanBP3 S126 by AKT1; this modification was previously shown to regulate the Ran gradient and nuclear transport [41] . Aside from these previously characterized NPC protein phosphosites, the specific functional effects of increased phosphorylation on the majority of NPC and associated proteins regulated by PI3K (10 out of 14) remain elusive. Nonetheless, our findings strongly suggest the likelihood of important roles for PI3K pathway activation in regulating mitotic NPC disassembly and nucleocytoplasmic transport. We were able to identify both classic and less-characterized networks that were regulated by the activation of PI3K pathway. Notably, in our global phosphoproteomic study, almost two-thirds of the regulated phosphoproteins whose phosphorylation patterns are correlated with PI3K/AKT activities could still not be mapped onto known kinase–substrate relationships or protein–protein interaction networks. It is worth noting that in addition to the well-known kinases such as AKTs and PDK1 involved in the canonical PI3K signalling, there are six different kinases also containing the pleckstrin homology domain that can bind to phosphatidylinositol 3,4,5-trisphosphate (PIP3). Among these kinases, four are non-receptor tyrosine kinases belonging to TEC tyrosine kinase family, namely TEC, TIK, BMX and BTK. Recent studies demonstrated that mutant PIK3CA could indeed activate BMX and directly phosphorylate STAT3 on Y705 (refs 42 , 43 ). In our study, we observed increased phosphorylation on S727 of STAT3 in our mutant Ex9-KI cells ( Supplementary Data 1 ) and treatment with J124 could reduce this phosphorylation. Besides these four tyrosine kinases, there are two serine/threonine kinases, TRIO and KALRN, which can also bind PIP3 through pleckstrin homology domains. However, exactly how these two kinases are regulated by and involved in PI3K signalling remains unknown. In this regard, it is important to note that we found that TRIO phosphorylation on S2455, S2476 and S2477 was closely associated with the activity of PI3K in mutant PIK3CA Ex9-KI cells. Further studies on these non-canonical PIP3-regulated kinases are necessary to interpret the profound alterations induced by mutant PIK3CA. The abundance of these novel PI3K-modulated phosphorylation events also indicates that our knowledge of this serine/threonine kinase-centred signalling cascade is still far from complete. Identification of novel AKT substrates Using the mass spectrometry-based phosphoproteomic approach, we identified 1,142 phosphopeptides (derived from 474 proteins) that were stringently correlated with PIK3CA and AKT activities (that is, more phosphorylated in knockin cells and less phosphorylated on J124 treatment). Of these, 358 phosphopeptides were derived from 204 proteins matching a minimal AKT substrate motif, R/KxxpS/T. When compared with the kinase substrate databases described above, 16 proteins were known AKT substrates ( Supplementary Data 7 ), including well-studied molecules in AKT signalling such as GSK3A, GSK3B, AKT1S1, EPHA2 and PFKFB2. However, ~92% (188 of the 204 proteins) were not previously reported as AKT substrates. It is indeed possible that although they contain the AKT substrate motif, other kinases in addition to AKT may also be able to phosphorylate these proteins on the same residues in vivo . A definitive way to assess this possibility is to use in vitro phosphorylation reactions to capture the direct phosphorylation targets of AKT. We employed a human protein microarray with 4,191 unique, full-length human proteins belonging to 12 major protein families to perform phosphorylation reactions with recombinant human AKT1 proteins in the presence of [γ- 32 P]-ATP (ref. 44 ). In comparison with a negative control reaction in which AKT1 was omitted, we identified 316 proteins ( Supplementary Data 8 ) that could be directly phosphorylated by AKT1 in vitro . To maximize the advantages of the two high-throughput proteomic approaches and to increase the confidence of identification of novel AKT substrates, we overlaid our mass spectrometry-based phosphoproteomic data with protein microarray-based data set and found six novel substrates that were regulated by PI3K in our PIK3CA mutation knockin cell line model and could also be directly phosphorylated in vitro by AKT1 in the protein microarray experiment ( Supplementary Fig. 5a ). To test whether these proteins were direct substrates of AKT1, we performed in vitro kinase reactions by mixing recombinant AKT1 with each of these six proteins (cortactin, TRIP10, PRKCD, PPP1R13L, EIF4B and C19ORF21) purified as glutathione S -transferase (GST) fusion proteins. All six proteins were phosphorylated by AKT1 ( Fig. 5a ), which provides solid evidence that these six proteins are bona fide AKT substrates. Interestingly, we identified a highly interconnected cluster containing PRKCD as a hub in our kinase–substrate and protein–protein interaction network analysis ( Fig. 4c ). This integrative analysis allowed us to confirm that the enrichment of PRKCD-centred network is probably the result of elevated phosphorylation of PRKCD by AKT1. 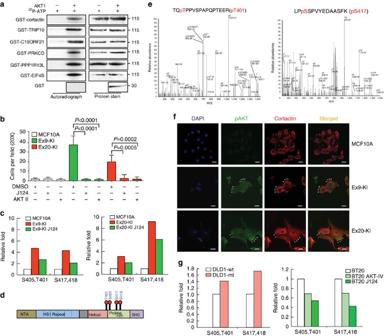Figure 5: Integrative analysis for identification of novel AKT substrates. (a)In vitroAKT1 kinase assays with indicated GST fusion proteins. Right panels: autoradiograph of32P-phosphorylated AKT1 substrates; left panels: Memcode staining of GST fusion proteins. (b) Matrigel migration/invasion assays for MCF10A, Ex9-KI and Ex20-KI cells treated with J124, AKT inhibitor IV or DMSO. Data are shown as mean±s.e.m. Mann–Whitney test was carried out to determine the statistical significance. The experiments were repeated twice. (c) Relative phosphorylation levels of cortactin phosphosites identified in SILAC-based phosphoproteomic analysis of Ex9-KI or Ex20-KI cells treated with or without J124 and parental MCF10A cells. (d) Domain structure of cortactin with phosphosites identified in this study. (e) Representative MS/MS spectra confirming phosphorylation of cortactin at T401 and S417 inin vitroAKT kinase–substrate assays followed by LC-MS/MS analysis. (f) Confocal immunofluorescence images of subcellular localization of cortactin (red) and pAKT(green) in MCF10A, Ex9-KI and Ex20-KI cells. Nuclei stained with DAPI. White arrows indicate the co-localization of cortactin and pAKT at peripheral region of lamellipodia. Scale bar, 20 μm. (g) Relative phosphorylation levels of cortactin in DLD1-wt and DLD1-mt cells (left), and in BT20 cells treated with or without J124 or AKT inhibitor IV (right). Figure 5: Integrative analysis for identification of novel AKT substrates. ( a ) In vitro AKT1 kinase assays with indicated GST fusion proteins. Right panels: autoradiograph of 32 P-phosphorylated AKT1 substrates; left panels: Memcode staining of GST fusion proteins. ( b ) Matrigel migration/invasion assays for MCF10A, Ex9-KI and Ex20-KI cells treated with J124, AKT inhibitor IV or DMSO. Data are shown as mean±s.e.m. Mann–Whitney test was carried out to determine the statistical significance. The experiments were repeated twice. ( c ) Relative phosphorylation levels of cortactin phosphosites identified in SILAC-based phosphoproteomic analysis of Ex9-KI or Ex20-KI cells treated with or without J124 and parental MCF10A cells. ( d ) Domain structure of cortactin with phosphosites identified in this study. ( e ) Representative MS/MS spectra confirming phosphorylation of cortactin at T401 and S417 in in vitro AKT kinase–substrate assays followed by LC-MS/MS analysis. ( f ) Confocal immunofluorescence images of subcellular localization of cortactin (red) and pAKT(green) in MCF10A, Ex9-KI and Ex20-KI cells. Nuclei stained with DAPI. White arrows indicate the co-localization of cortactin and pAKT at peripheral region of lamellipodia. Scale bar, 20 μm. ( g ) Relative phosphorylation levels of cortactin in DLD1-wt and DLD1-mt cells (left), and in BT20 cells treated with or without J124 or AKT inhibitor IV (right). Full size image Cortactin is a novel AKT substrate regulating cell invasion We have previously demonstrated that PIK3CA mutations can enhance cell migration and invasion of cancer cells [9] . Analysis of the phosphorylation data revealed enrichment of signalling pathways regulating cell migration and cytoskeletal rearrangement in PIK3CA mutant knockin cells ( Fig. 2g and Supplementary Fig. 2e ). To investigate the effects of these phosphorylation-increased pathways in non-tumorigenic breast epithelial cells containing mutant alleles of PIK3CA , we employed matrigel-coated Boyden chamber assays to evaluate their invasive abilities. The results revealed that Ex9-KI and Ex20-KI cells could indeed penetrate matrigel to a much greater extent than the parental MCF10A cells. Moreover, the invasive ability enhanced by activation of PIK3CA could be dramatically attenuated by treatment with the PIK3CA inhibitor, J124, as well as by the AKT inhibitor IV ( Fig. 5b ). Of the six confirmed novel direct substrates of AKT substrates, cortactin ( CTTN ) was of special interest because it is a component of the enriched pathways related to cell motility and cytoskeleton ( Fig. 2g and Supplementary Fig. 2e ). Cortactin is a key branched actin regulator that regulates cell motility and transduces signals from the cell membrane to cytoskeletal proteins. It is frequently overexpressed in advanced cancers and enhances cancer cell migration and invasion [45] , and ectopic overexpression of cortactin in head and neck squamous cell carcinoma cell lines has been reported to increase AKT activity [46] . As a key regulator of actin branching, the activity of cortactin activity is modulated by multiple kinases, including tyrosine kinases SRC and FYN, and serine/threonine kinases ERK1/2 and PAK1 (ref. 45 ). Our phosphoproteomic studies revealed that phosphorylation of cortactin at S405/T401 and S417/S418 was regulated by the PI3K-AKT pathway ( Fig. 5c ). These four phosphorylation sites are located within or close to the proline-rich domain of cortactin ( Fig. 5d ), which contains many sites of tyrosine and serine phosphorylation regulated by different kinases [45] . For instance, ERK kinase has been shown to phosphorylate cortactin on S405 and S418 (ref. 47 ). To confirm that AKT1 can also directly phosphorylate cortactin, we performed LC-MS/MS analysis of purified cortactin incubated in vitro with AKT1. This experiment confirmed that AKT is able to directly phosphorylate all four sites (S405/T401 and S417/S418) of cortactin ( Fig. 5e and Supplementary Fig. 6a,b ). To investigate whether cortactin and AKT interact in vivo , we performed immunofluorescence staining to examine the localization patterns of cortactin and phosphorylated AKT (pS473). As demonstrated in Fig. 5f , we could clearly observe the co-localization of cortactin and phosphorylated AKT in Ex9-KI and Ex20-KI cells. It is worth noting that the co-localization pattern was concentrated at the peripheral region of lamellipodia in Ex9-KI and Ex20-KI cells. We also performed immunofluorescence staining to examine the interaction between cortactin and its known partners in MCF10A, Ex9-KI and Ex20-KI cells. Cortactin largely co-localized with its interaction partners WASP, NCK1 and cofilin in all tested cell lines ( Supplementary Fig. 6c ). The co-localization patterns of cortactin and cofilin, NCK1 and WASP in peripheral membrane structures were only detected in Ex9-KI and Ex20-KI cells with PIK3CA mutations ( Supplementary Fig. 6c ). To test whether phosphorylation of cortactin could also be regulated by AKT1 in other cells with alterations in the PI3K signalling pathway, we used another isogenic cell line pair derived from the colorectal cancer cell line DLD1 (ref. 9 ). The parental line contained one wt PIK3CA allele and one mutant allele (E545K), and the two derivatives were created by homologous recombination so that one contained only the wt PIK3CA allele (DLD1-wt), while the other contained only the mutant allele (DLD1-mt). LC-MS/MS analysis was performed on anti-cortactin immunoprecipitates from cell lysates extracted from SILAC-labelled DLD1-wt (light) and DLD1-mt (heavy) cells ( Supplementary Fig. 5b,c ). This experiment showed that DLD1-mt cells had higher levels of phosphorylation of cortactin than DLD1-wt cells ( Fig. 5g , left panel). We also investigated a breast cancer cell line, BT20, harbouring mutant PIK3CA alleles [48] . Cell lysates from SILAC heavy-labelled BT20 cells treated with J124 or AKT inhibitor IV (AKT-IV) were mixed with untreated cells, then subjected to immunoprecipitation with anti-cortactin antibody ( Supplementary Fig. 5b ). LC-MS/MS analysis of immunoprecipitated cortactin again revealed that phosphorylation levels of cortactin were substantially reduced in BT20 cells treated with either J124 or AKT inhibitor IV ( Fig. 5g , right panel). To further characterize the role of cortactin in promoting migration/invasion of PIK3CA mutant cells, we first employed small interfering RNA (siRNA) to knockdown cortactin expression in MCF10A, Ex9-KI and Ex20-KI cells ( Fig. 6a top panel). We found that knockdown of cortactin significantly reduced the invasive ability of PIK3CA mutant knockin cells ( Fig. 6a ). A similar suppression of invasion was observed in DLD1-mt and BT20 cells after knockdown of cortactin expression ( Fig. 6b,c ). We next wanted to determine the phosphorylation effect of cortactin on its function. Cortactin has been shown to possess three alternatively spliced isoforms encoding three different proteins that are 550, 513 or 634 amino acids long. To identify the predominant isoform(s) expressed in MCF10A cells, we conducted a database search against transcript databases in addition to carrying out reverse transcriptase–PCR using primers that could distinguish specific isoforms ( Supplementary Fig. 6d ). We found that transcripts of isoforms A and B, but not C, were detectable in MCF10A and mutant PIK3CA knockin cells. Thus, we cloned both of these isoforms into a retroviral expression vector and carried out site-directed mutagenesis to alter all four detected AKT1 phosphorylation sites (S405A, T401A, S417A and S418A). Wild-type and mutant versions of both cortactin isoforms (A and B) were stably expressed in parental MCF10A, Ex9-KI and Ex20-KI cells, as confirmed by western blot analysis ( Fig. 6d ). Boyden chamber assays were employed to examine the effects of cortactin phosphorylation on cell migration and invasion where we found that overexpression of wt isoforms A and B promoted cell migration and invasion ( Fig. 6d ), and this enhanced invasive capacity could be reduced by the treatment of AKT inhibitor ( Supplementary Fig. 6e ), suggesting that AKT-mediated phosphorylation of cortactin contributes to the invasive ability induced by overexpression of cortactin. In contrast, overexpression of the mutant isoforms that could not be phosphorylated by AKT1 did not enhance, and perhaps even suppressed the migration and invasive ability of the cells ( Fig. 6d ). Similar effects were observed in BT20 cells bearing PIK3CA mutations ( Fig. 6e ). 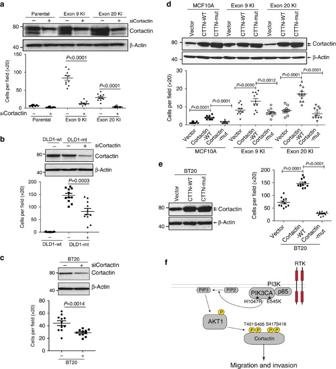Figure 6: AKT1-mediated phosphorylation on cortactin is important for migration/invasion induced by activation of PI3K. (a) Top panel: western blotting with cortactin antibody to assess the knockdown efficiency of siRNA targeting cortactin in MCF10A, Ex9-KI and Ex20-KI cells. β-Actin served as loading control. Bottom panel: matrigel-coated Boyden chamber assays for the assessment of the migration/invasion ability of cells with indicated siRNA knockdown. (b,c) siRNA knockdown of cortactin in DLD1-mt (b) and BT20 cells (c). Top panels: western blotting of cortactin and β-actin; bottom panels: Boyden chamber assays of indicated cell lines. (d,e) Migration/invasion assays for MCF10A, Ex9-KI, Ex20-KI and BT20 cells overexpressing wild-type cortactin isoform A and B (cortactin-wt) and phosphosite-mutated cortactin isoform A and B (cortactin-mut). Top panels: western blottings of overexpressed cortactin; bottom panels: migration/invasion assays of indicated cells. (f) A proposed model of enhancing invasiveness by oncogenic activation of PI3K-AKT signalling cascades and phosphorylation of cortactin. (a–e) Data are shown as mean±s.e.m. Mann–Whitney test was carried out to determine the statistical significance. These experiments were repeated at least twice. Figure 6: AKT1-mediated phosphorylation on cortactin is important for migration/invasion induced by activation of PI3K. ( a ) Top panel: western blotting with cortactin antibody to assess the knockdown efficiency of siRNA targeting cortactin in MCF10A, Ex9-KI and Ex20-KI cells. β-Actin served as loading control. Bottom panel: matrigel-coated Boyden chamber assays for the assessment of the migration/invasion ability of cells with indicated siRNA knockdown. ( b , c ) siRNA knockdown of cortactin in DLD1-mt ( b ) and BT20 cells ( c ). Top panels: western blotting of cortactin and β-actin; bottom panels: Boyden chamber assays of indicated cell lines. ( d , e ) Migration/invasion assays for MCF10A, Ex9-KI, Ex20-KI and BT20 cells overexpressing wild-type cortactin isoform A and B (cortactin-wt) and phosphosite-mutated cortactin isoform A and B (cortactin-mut). Top panels: western blottings of overexpressed cortactin; bottom panels: migration/invasion assays of indicated cells. ( f ) A proposed model of enhancing invasiveness by oncogenic activation of PI3K-AKT signalling cascades and phosphorylation of cortactin. ( a – e ) Data are shown as mean±s.e.m. Mann–Whitney test was carried out to determine the statistical significance. These experiments were repeated at least twice. Full size image These studies, in aggregate, provide strong evidence that mutations of PIK3CA enhance the migration and invasiveness of cells through the activation of AKT and the subsequent phosphorylation of cortactin ( Fig. 6f ). Oncogenic mutations in PIK3CA gene have been reported in many human cancer types. Using a gene targeting approach to knockout either wt or mutant PIK3CA alleles in colorectal cancer cell lines, Samuels et al. [9] have previously demonstrated that mutant PIK3CA selectively regulated the phosphorylation level of AKT and its downstream transcription factors FKHR and FKHRL1. However, a comprehensive and quantitative analysis of how PIK3CA mutants globally impact signalling networks and consequently transform epithelial cells has not yet been reported. In this study, we employed an isogenic model system to characterize the signalling alterations induced by the knockin of two hotspot oncogenic PIK3CA mutations (E545K or H1047R) in a spontaneously immortalized non-tumorigenic breast epithelial cell line, MCF10A. This system can model breast epithelial cell malignancy induced by PIK3CA mutations. Using this unique model system, we applied a comprehensive phosphoproteomic analysis to discern and quantify global activation of phosphorylation-mediated signalling networks caused by these two PIK3CA mutations. Based on our phosphoproteomic analysis, it is possible that the elevation of the phosphorylation of some proteins resulted from the increased protein expression or the accumulation of both increased protein abundance and phosphorylation level. More importantly, we also observed phosphorylation of more than a thousand peptides from 474 proteins to be increased in PIK3CA mutant knockin cells and reduced on the short-term treatment with the PIK3CA inhibitor, J124. These changes are probably regulated by phosphorylation induced by mutant PIK3CA and not through the increase of protein abundance. Among these phosphorylation-increased proteins, only a fraction (208/474) has been reported to be involved in signalling networks related to the canonical PI3K-AKT signalling pathway. To our knowledge, this study provides the most comprehensive survey of quantified signalling perturbations in phosphorylation resulting from oncogenic activation of mutant PIK3CA . These newly identified signalling events should increase our understanding of the oncogenic effects resulting from mutations in PIK3CA gene, especially for development of novel therapeutic strategies for cancers with PIK3CA mutations. From this data set, we were able to demonstrate increased phosphorylation of many key enzymes involved in important signalling networks and cellular processes in this predominantly serine/threonine kinase-driven signalling network. For instance, we have demonstrated increased phosphorylation of several key tyrosine kinases ( Fig. 3a ). In addition, we identified modulation of phosphorylation of an AKT substrate, ACLY, which is the primary enzyme synthesizing cytosolic acetyl CoA. Acetyl CoA is the essential precursor for fatty acids, mevalonate synthesis [49] and a major source for protein acetylation reactions, including histone acetylation [50] . Phosphorylation-induced activation of ACLY by oncogenic mutation of PIK3CA could have the potential to enhance de novo fatty acid synthesis and also to globally regulate chromatin architecture and gene transcription. We also observed increased phosphorylation of ubiquitin protein E3 ligase (UBR4, ubiquitin protein ligase E3 component n-recognin 4) and several ubiquitin-specific peptidases (USP10, USP24 and USP43) in mutant PIK3CA knockin cells and the increase phosphorylation was diminished on J124 treatment. Some of these (UBR4, USP10 and USP24) were reported to be involved in oncogenic transformation of epithelial cells [51] , [52] , [53] . These data suggest that PIK3CA oncogenic mutations not only globally modulate protein phosphorylation but can also potentially regulate multiple other post-translational modifications via the cross-talk between kinases and other enzymes. Our integrated approach to identify kinase substrates by combining two high-throughput proteomic platforms—mass spectrometry-based phosphoproteomics and protein microarray-based kinase assays—enabled us to identify six novel AKT substrates. Functional studies confirmed that phosphorylation of one novel substrate, cortactin, is critical for migration/invasion induced by oncogenic activation of PI3K. Similar approaches employing high-throughput proteomic technology-based strategies can be applied to understand other cancer signalling pathways in a systematic manner. In summary, mutant PI3K-induced signalling events uncovered by our phosphoproteomic approaches along with the newly identified AKT1 substrates should be invaluable for research as well as clinical studies involving development of novel targeted therapies. Cell culture and reagents Cell lines were grown in 5% CO 2 at 37 °C. The breast epithelial cell line MCF-10A was purchased from American Type Culture Collection, and its PIK3CA mutant knockin cell lines, Ex9-KI and Ex20-KI were previously generated using gene targeting method [8] . The cells were cultured in DMEM/F12 (1:1) supplemented with 5% horse serum, 20 ng ml −1 epidermal growth factor (EGF) for MCF10A parental cells and 0.2 ng ml −1 EGF for knockin cells. In addition, 10 μg ml −1 insulin (Roche), 0.5 μg ml −1 hydrocortisone (Sigma) and 100 ng ml −1 cholera toxin (Sigma) were supplemented for all cells. To label cells with stable isotopic amino acids, MCF10A and PIK3CA mutation knockin cells were propagated in DMEM/F12 SILAC media with corresponding complete supplements, but deficient in both L -lysine and L -arginine (Thermo Fisher Scientific) and supplemented with light lysine (K) and arginine (R) for light, 2 H 4 -K and 13 C 6 -R for medium state, and 13 C 6 15 N 2 -K and 13 C 6 15 N 4 -R for heavy state labelling (Cambridge Isotope Laboratories). Cells were seeded at 80% confluence in 5% horse serum DMEM/F12 basal media overnight. Cells were pretreated for 3 h with 0.2 ng ml −1 EGF that is close to the physiological concentration of EGF in serum [54] and followed by 30-min treatment of 500 ng ml −1 J124 or 0.05% dimethyl sulphoxide (DMSO) as vehicle control before harvesting. Before harvesting, cells were checked under microscope to ensure the proper confluence and healthy status. The phase-contrast images of cells before harvesting were shown in Supplementary Fig. 1a . Immunoblotting and siRNA knockdown Cells were harvested and lysed in modified RIPA buffer (50 mM Tris–HCl, pH 7.4, 150 mM NaCl, 1 mm EDTA, 1% Nonidet P-40, 0.25% sodium deoxycholate and 1 mM sodium orthovanadate in the presence of protease inhibitors). Whole-cell protein extracts were denatured and separated in NuPAGE gels (Invitrogen), transferred to nitrocellulose membranes and probed with primary and horseradish peroxidase-conjugated secondary antibodies. Anti-p44/p42 MAPK (9102: 1:1,000), anti-phospho-p44/p42 MAPK-Thr202/Tyr204 (9106: 1:1,000), anti-AKT (9272: 1:1,000), anti-pAKT-Ser473/Thr308 (9271, 2965: 1:1,000), anti-ACLY (4332: 1:1,000), anti-pACLY-Ser544 (4331: 1:1,000), anti-pGSK3β-Ser9 (5538: 1:1,000), anti-GSK3β (9832:1:1,000) and anti-pEPHA2-Ser897 (6347: 1:1,000) were purchased from Cell Signaling Technology. Other antibodies used are anti-EPHA2 (3625: 1:1,000) from Epitomics and anti-β-actin (A5316:1:5,000) from Sigma. Full scans of western blottings are provided in Supplementary Fig. 7 . siRNA (50 nM) (5′-CACCAGGAGCAUAUCAACAUA-3′) targeting cortactin (Qiagen) was used for transfections with RNAiMax (Invitrogene). Cells were harvested 48 h post transfection for assessing knockdown efficiency or other follow-up experiments. Site-directed mutagenesis and stable overexpression Full-length cortactin CDS plasmids for isoform A and B were purchased from DNA Resource Core (Harvard) and subcloned into pBABE-puro vector. Site-directed mutagenesis for cortactin mutants was performed with QuikChange Site-Directed Mutagenesis Kit (Agilent). HEK293T cells were used for retroviral package. Briefly, pBABE-cortactin wt, mutant expression plasmids or control empty vector plasmids were co-transfected with pCL-Ampho (Imagenex) packing plasmid. Virus supernatants were collected and used for infection of MCF10A and knockin cells. Infected cells were then selected by 0.5 μg ml −1 puromycin to obtain cells stably expressing cortactin proteins. Trypsin digestion Cell lysates were prepared in urea lysis buffer containing 20 mM HEPES pH 8.0, 9 M urea, 1 mM sodium orthovanadate, 2.5 mM sodium pyrophosphate, 1 mM β-glycerophosphate and 5 mM sodium fluoride. The lysates were sonicated and cleared by centrifugation at 3,000 g at 4 °C for 10 min Protein estimation was carried out using BCA protein assays. Equal amount of protein from three SILAC-labelled states were mixed, reduced with 5 mM dithiothreitol and alkylated with 10 mM iodoacetamide. Lysates were diluted to <2 M urea final concentration in 20 mM HEPES (pH 8.0) and incubated with L-1-tosylamido-2-phenylethyl chloromethyl ketone (TPCK)-treated trypsin at 25 °C overnight. The reaction was quenched using 1% trifluoroacetic acid. The protein digest was desalted using C 18 reverse phase column (Waters, UK) and eluted peptides were lyophilized and subjected to phosphopeptide enrichment. TiO 2 -based phosphopeptide enrichment Peptides were fractionated by strong cation exchange (SCX) chromatography as described earlier [55] . Briefly, 10 mg of lyophilized peptides mixture was resuspended in 1 ml of SCX solvent A (5 mM KH 2 PO 4 pH 2.7, 30% ACN) and were separated on a PolySULPHOETHYL A column (5 μm, 200 Å, 200 × 9.4 mm; PolyLC Inc., Columbia, MD) with an increasing gradient of SCX solvent B (5 mM KH 2 PO 4 pH 2.7, 30% ACN, 350 mM KCl) on an Agilent 1100 HPLC system. In total, 15 fractions were collected. Each fraction was subjected to TiO 2 -based phosphopeptide enrichment as described earlier [56] . Briefly, TiO 2 beads were incubated with DHB solution (80% ACN, 1% TFA, 3% 2,5-dihydroxybenzoic acid (DHB)) for 4 h at room temperature. Each fraction was resuspended in DHB solution and incubated with pretreated TiO 2 beads (5 mg). Phosphopeptide-bound TiO2 beads were washed three times with DHB solution and twice with 40% ACN. Peptides were eluted three times with 40 μl of 2% ammonia into 10 μl of 20% TFA. Liquid chromatography–tandem mass spectrometry LC-MS/MS analysis of enriched phosphopeptides was carried out using a reverse-phase LC system interfaced with an LTQ-Orbitrap Velos mass spectrometer (Thermo Fisher Scientific). The peptides were loaded onto an analytical column (10 cm × 75 μm, Magic C18 AQ 5 μm, 120 Å) in 0.1% formic acid and eluted with a linear gradient from 5% to 60% ACN in 90 min. Precursor scans fourier transform mass spectrometry (FTMS) were acquired in the range of 350–1,700 m/z at 60,000 resolution at 400 m/z on an Orbitrap analyser. Ten most abundant precursor ions from a survey scan were selected for Higher-energy collisional dissociation (HCD) fragmentation (isolation width of 1.90 m/z ; 35% normalized collision energy and activation time of 0.1 ms were allowed) and MS2 spectra were acquired at 15,000 resolution at 400 m/z on the Orbitrap analyser. Mass spectrometry data analysis Proteome Discoverer (v 1.3; Thermo Fisher Scientific) suite was used for quantitation and database searches. The MS/MS data were searched using Mascot (Version 2.2.0) and SEQUEST search algorithms against a Human RefSeq database (v 46 containing 33,249 entries) supplemented with frequently observed contaminants. For both algorithms, the search parameters included the following: (i) a maximum of one missed cleavage; (ii) carbamidomethylation of cysteine as a fixed modification; (iii) amino-terminal acetylation; (iii) oxidation at methionineand; (iv) phosphorylation at serine, threonine and tyrosine; and (v) SILAC labelling 13 C 6 , 15 N 2 -lysine, 2 H 4 -lysine, 13 C 6 -arginine and 13 C 6, 15 N 2 -arginine as variable modifications. The MS tolerance was set at 10 p.p.m. and MS/MS tolerance to 0.1 Da. Score cutoff value was set to 0.01 false discovery rate at the peptide level. The probability of phosphorylation for each Ser/Thr/Tyr site on each peptide was calculated by the PhosphoRS algorithm [57] . We averaged the intensities of phosphopeptides identified from the forward and reverse experimental groups. We chose a 1.5-fold cutoff value to consider peptides as phosphorylation increased and a 0.67-fold for peptides to be considered as phosphorylation decreased. This threshold was chosen because we observed that AKT phosphorylation increased by 1.53-fold in PIK3CA mutant knockin cells. Many of the known phosphorylation sites of AKT substrates were found to range between 1.5- and 2-fold in the knock-in cell lines compared with the parental cells. Among these were BAD S75 (1.82), CTNNB1 S552 (1.62), HSPB1 S82 (1.81), PDCD4 S457 (1.50), PEA15 S116 (1.60), RANBP3 S126 (1.96) and YAP1 S127 (1.65). To identify and plot the differentially regulated phosphopeptides, we averaged the intensity of each phosphopeptide detected from MCF10A, PIK3CA mutant knockin cells and knockin cells treated with PIK3CA inhibitor, J124. The relative ratio was calculated by dividing the intensity of each phosphorylated peptide over the average intensity of the corresponding peptide and used for plot. The MS proteomics data have been deposited to the ProteomeXchange Consortium ( http://proteomecentral.proteomexchange.org ) via the PRIDE partner repository. Motif analysis The surrounding sequence (seven amino acid residues on either side) for each identified phosphorylation site was extracted from the RefSeq database. For phosphorylation sites that were localized at the region of the N- or carboxy termini, the surrounding sequence could not be extended in this manner were excluded from further motif analysis. The motif-x algorithm ( http://motif-x.med.harvard.edu ) was used to extract motifs. The significance threshold was set to P <1e−3. The minimum occurrence of motif was set to 20 for pSer peptides against an IPI Human proteome background. The NetworKIN ( http://networkin.info ) tool was used to identify predicted protein kinases for all phosphosites as substrates. These were further classified based on motifs identified by motif-X. Kinase–substrate and protein interaction network analysis Three major kinase substrate databases, HPRD ( www.hprd.org ), PhosphositePlus ( www.phosphosite.org ) and Phospho.ELM ( http://phospho.elm.eu.org ), and one comprehensive protein–protein interaction database MIMI ( http://mimi.ncibi.org ) were merged based on kinase–substrate and protein–protein interaction pairs. If the protein pairs had both kinase–substrate in interaction partnerships, only kinase–substrate relationship was retained. We mapped 474 proteins whose phosphorylation levels were directly correlated with PI3K activity, with the merged database. Only kinase–substrate and protein interactions between the proteins belonging to the searched data set were selected, thereby excluding external candidates. The network was visualized by Cytoscape in the mode of force-directed layout. A graph theoretical clustering algorithm, molecular complex detection [35] was used to identify densely connected clusters. In vitro kinase assays GST fusion proteins were generated in yeast or bacterial systems and purified with Glutathione–Sepharose beads. The GST fusion proteins were pretreated with lambda phosphatase (NEB) at 30 °C for 30 min and incubated at 60 °C for another 30 min to inactivate any phosphatase activity. Pre-treated GST fusion proteins were mixed with 32 P-ATP (250 μCi) and with or without 100 ng AKT1 for 30 min at 30 °C. The samples were resolved by SDS–PAGE and the proteins were transferred onto nitrocellulose membranes. Phosphorylated and total proteins were visualized by autoradiography or MemCode staining (Thermo), respectively. To examine AKT1-induced phosphorylation sites, cortactin–GST fusion proteins were incubated with 1 mM ATP in the presence or absence of AKT1 at 30 °C for 30 min. The samples were then resolved by SDS–PAGE and visualized by Coomassie blue staining. Gel bands were excised and digested with tryspin. Tryptic peptides were extracted and analysed on an LTQ-Orbitrap Elite mass spectrometer. MS data were searched against Human RefSeq with Sequest and Mascot algorithms. Matrigel invasion assays Cells were trypsinized and 5 × 10 4 cells were seeded onto Biocoat matrigel invasion chambers (BD Biosciences) in 1% horse serum in DMEM/F12 medium for MCF10A cells and serum-free media for DLD1 and BT20 cells. Complete medium was added in the lower chamber as chemoattractant. After 24 h, the filter membranes were stained with DAPI (4',6-diamidino-2-phenylindole) (Invitrogen) and the number of cells that penetrated through the matrigel and membrane was counted in ten randomly selected view fields at × 20 magnification. Immunofluorescence analysis Cells were seeded in 5% DMEM-F12 medium with 5% horse serum overnight and treated with 0.2 ng ml −1 EGF for three hours before fixation with 4% paraformaldehyde. Fixed cells were permeabilized with 0.05% Triton X-100 and blocked with 3% bovine serum albumin in PBS. Cortactin was visualized with by immunofluorescence (IF) with anti-cortactin mAb 4F11 (05–180; 1:500) from Millipore and Alexa Fluor 568-labelled goat anti-mouse IgG secondary antibody (A11031; 1:1,000) from Invitrogen. IF assays were also performed with rabbit monoclonal anti-phosphorylated AKT (pS473) (4058: 1:200) antibody from Cell Signaling Technology, and rabbit polyclonal antibodies against WASP (SC-8350: 1:250) from Santa Cruz, NCK1 (ab23120: 1:200) from Abcam and cofilin (SC-33779:1:200) from Santa Cruz, followed by Alexa Fluor 488-labelled goat anti-rabbit IgG secondary antibody (A11034, 1:1,000) from Invitrogen. The nuclei were stained with SlowFade Gold Antifade Mountant with DAPI (S36938) from Life Technologies. IF analysis was carried out using a LSM710 confocal laser scanning microscope (Carl Zeiss). Immunoprecipitation SILAC-labelled DLD1-wt (light) and DLD1-mt (heavy) cells and SILAC-labelled BT20 cells treated with DMSO (light) or J124 (heavy) were lysed with modified RIPA buffer. Equal amount of the protein lysates from DLD1-wt (light) and DLD1-mt (heavy), or BT20 DMSO-treated (light) and BT20 J124-treated (heavy) cells were mixed and followed by immunoprecipitation with cortactin antibody 4F11 (05–180, Millipore). The precipitated proteins were subjected to SDS–PAGE and stained with Coomassie brilliant blue R250. The cortactin band was excised for MS analysis. Reverse transcriptase–PCR Total RNA was extracted with TRIZOL reagent (Invitrogen) and complementary DNA synthesized using SuperScript II Reverse Transcriptase kit (Invitrogen) according to the manufacturer’s instructions. Forward: 5′-GAGCGCGGTGGGCTTCGACTAC-3′ and reverse: 5′-CTCCGCCTTCCGCCTGTCCTCC-3′ primers were used to amplify isoform-specific region to distinguish isoform A from isoform B and C. Forward: 5′-GGGCCACTATCCCGCAGAGGAC-3′ and reverse: 5′-GACTGCACTTGATGGGCACGAG-3′ primers were used to amplify a specific region to distinguish isoform C from isoforms A and B ( Supplementary Fig. 6d ). Accession codes: The mass spectrometry proteomics data have been deposited to the ProteomeXchange Consortium ( http://proteomecentral.proteomexchange.org ) via the PRIDE partner repository with the data set identifier PXD000599. How to cite this article: Wu, X. et al. Activation of diverse signaling pathways by oncogenic PIK3CA mutations. Nat. Commun. 5:4961 doi: 10.1038/ncomms5961 (2014).